Activin enhances skin tumourigenesis and malignant progression by inducing a pro-tumourigenic immune cell response Activin is an important orchestrator of wound repair, but its potential role in skin carcinogenesis has not been addressed. Here we show using different types of genetically modified mice that enhanced levels of activin in the skin promote skin tumour formation and their malignant progression through induction of a pro-tumourigenic microenvironment. This includes accumulation of tumour-promoting Langerhans cells and regulatory T cells in the epidermis. Furthermore, activin inhibits proliferation of tumour-suppressive epidermal γδ T cells, resulting in their progressive loss during tumour promotion. An increase in activin expression was also found in human cutaneous basal and squamous cell carcinomas when compared with control tissue. These findings highlight the parallels between wound healing and cancer, and suggest inhibition of activin action as a promising strategy for the treatment of cancers overexpressing this factor. There are remarkable similarities between wound healing and cancer [1] , and the presence of a 'wound healing gene expression signature' is a hallmark of highly malignant carcinomas [2] . Therefore, it is of particular interest to identify wound-regulated genes and to characterize their functions in cancer development and progression. Major orchestrators of wound repair are activins, which belong to the transforming growth factor (TGF)-β superfamily of growth and differentiation factors. The most abundant activin variant is activin A, the homodimer formed by two βA subunits. Activins exert their biological effects through activation of transmembrane serine/threonine kinase receptors. Binding to a type II activin receptor (ActRII or ActRIIB) leads to the phosphorylation and activation of a type I activin receptor (ActRIB, also known as Alk4, ActRIA=Alk2 or ActRIC=Alk7). This activates the canonical signalling pathway via Smad proteins, or, alternatively, mitogen-activated kinase pathways [3] . Activins were initially described as reproductive hormones, but they also have important functions in development, tissue homoeostasis and repair [4] . Furthermore, abnormalities in activin receptor expression and/or signalling are associated with various human diseases, including cancer [5] . We previously showed a strong increase in activin βA expression in healing skin wounds [6] . This is functionally relevant, as transgenic mice overexpressing the activin antagonist follistatin in keratinocytes showed delayed wound repair [7] , whereas overexpression of activin βA in keratinocytes strongly accelerated the healing process. However, healed wounds of activin-overexpressing mice had a hyperproliferative neo-epidermis (ref. 8 , and M.A. and S.W. unpublished results). Therefore, we speculated about a role of activin in the pathogenesis of skin cancer. Few functional studies have addressed the role of activin in malignancy, and pro- or anti-tumourigenic effects of activin have been reported, depending on the tissue and the type of cancer [9] , [10] , [11] . Most of these data were obtained with xenograft models in immunocompromised hosts, whereas a potential role of the immunomodulatory actions of activin [12] in the pathogenesis of cancer has not been addressed. In this study, we identified a novel and unexpected function of activin in the pathogenesis of non-melanoma skin cancer that is mediated through its effect on different epidermal immune cells. Activin promotes skin tumourigenesis in mice To determine a potential role of activin in skin carcinogenesis, we used transgenic mice expressing activin βA in keratinocytes under control of the keratin 14 (K14) promoter (Act mice) [8] . They secrete high levels of activin A, which can act on keratinocytes directly but also on stromal cells due to the high diffusibility of activin A [13] . This is reflected by the 30-fold increase in activin A levels in skin lysates and the 200-fold increase in the serum compared with wild-type (wt) animals ( Supplementary Fig. S1 ). Expression of high levels of activin A by keratinocytes did not interfere with the growth inhibitory effect of TGF-β on keratinocytes ( Supplementary Fig. S1 ). Most importantly, the back skin of these mice did not reveal any histological abnormalities, and keratinocyte proliferation in normal back skin epidermis was not affected by the enhanced levels of activin [8] . Act mice as well as sex- and age-matched wt littermates were subjected to a two-stage chemical skin carcinogenesis protocol, where tumours are induced by topical treatment of the back skin with 7,12-dimethylbenz[a]anthracene (DMBA), followed by weekly treatment with 12-O-tetradecanoylphorbol 13-acetate (TPA) [14] , [15] . 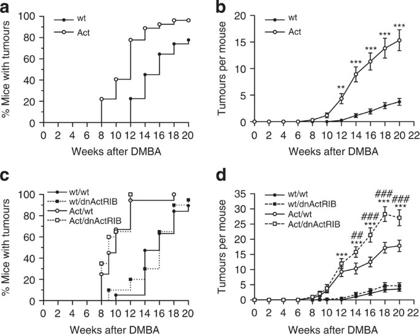Figure 1: Activin promotes chemically induced skin tumourigenesis in mice via action on stromal cells. (a,b) Kinetics of tumour incidence (a) or multiplicity (b) observed in experiment I (Table 1).N=31 wild-type (wt) mice;N=29 activin-transgenic (Act) mice. (c,d) Kinetics of tumour incidence (c) and multiplicity (d) in experiment III.N=18 mice per genotype. Kaplan–Meier survival curves are shown in (a) and (c); mean±s.e.m. are shown in (b) and (d); **P<0.01, ***P<0.001 for the comparison between wt/wt and Act/wt mice; ##P<0.01, ###P<0.001 for the comparison between Act/wt and Act/dnActRIB mice (two-way repeated measures ANOVA and Bonferroni post-test). A remarkable pro-tumourigenic effect of activin was observed in three independent experiments with mice of different genetic background (experiments I–III, Table 1 ) as reflected by the earlier appearance of papillomas and the strong increase in the percentage of mice with tumours (tumour incidence) and in the number of tumours per mouse (tumour multiplicity) ( Fig. 1a,b; Supplementary Fig. S2 ). Mice treated only with DMBA or TPA did not develop tumours, demonstrating that both a mutagenic insult and a proliferative stimulus are required. This is consistent with the finding that wounding alone did not induce tumourigenesis in control or Act mice (M.A. and S.W., unpublished results). Table 1 Summary of carcinogenesis experiments. Full size table Figure 1: Activin promotes chemically induced skin tumourigenesis in mice via action on stromal cells. ( a , b ) Kinetics of tumour incidence ( a ) or multiplicity ( b ) observed in experiment I ( Table 1 ). N =31 wild-type (wt) mice; N =29 activin-transgenic (Act) mice. ( c , d ) Kinetics of tumour incidence ( c ) and multiplicity ( d ) in experiment III. N =18 mice per genotype. Kaplan–Meier survival curves are shown in ( a ) and ( c ); mean±s.e.m. are shown in ( b ) and ( d ); ** P <0.01, *** P <0.001 for the comparison between wt/wt and Act/wt mice; ## P <0.01, ### P <0.001 for the comparison between Act/wt and Act/dnActRIB mice (two-way repeated measures ANOVA and Bonferroni post-test). Full size image Activin induces skin carcinogenesis via the stroma To determine if activin stimulates skin tumourigenesis through autocrine activation of keratinocytes and/or through paracrine/endocrine activation of stromal (mesenchymal or immune) cells, we used transgenic mice expressing a dominant-negative mutant of ActRIB (Alk4) in keratinocytes under control of the K14 promoter (dnActRIB mice) and mated them with Act mice. dnActRIB lacks the complete intracellular kinase domain, and through formation of non-functional heterodimers with type II activin receptors it efficiently blocks activin but not TGF-β signalling [16] . This approach was chosen, as keratinocytes express multiple activin receptors [6] , which are all inhibited by dnActRIB. The dnActRIB mice have no obvious phenotypic abnormalities under non-challenged conditions [16] , and the dnActRIB transgene neither affected expression of the activin βA transgene nor the bioavailability of the recombinant activin A (data not shown and Supplementary Fig. S1 ). Therefore, in Act/dnActRIB mice, the highly diffusible, recombinant activin can activate all cells in the skin, but its effect on keratinocytes is antagonized by dnActRIB expressed by these cells. The functionality of dnActRIB in the double-transgenic mice had previously been demonstrated [16] and was further verified by analysis of S100A8 and S100A9 expression. Thus, we had previously shown a strongly increased expression of these cytokines in the hyperthickened tail epidermis of Act mice [17] . We verified this increase with new mice (250-fold) and found that it was almost completely suppressed (>90%) in Act/dnActRIB mice (data not shown). We performed a two-stage chemical skin carcinogenesis study with the F1 progeny of dnActRIB and Act mice (experiment III, Table 1 ). The latency period and tumour incidence of the activin-overexpressing mice were not affected by dnActRIB ( Fig. 1c ), but the tumour multiplicity was significantly increased in the double-transgenic mice as compared with Act single-transgenic animals ( Fig. 1d ). This finding points to the existence of a tumour-inhibitory effect of activin A, which is mediated via keratinocytes and therefore affected by dnActRIB and which depends on the presence of high levels of activin. However, the potent pro-tumourigenic effect seems to be predominantly mediated via the stroma. Activin promotes tumour malignancy The vast majority of the tumours collected 20 weeks after initiation were papillomas ( Fig. 2a ). There was no difference in tumour cell proliferation and apoptosis between genotypes ( Supplementary Fig. S2 and data not shown), but several tumours in activin-overexpressing mice already contained sites of high-grade dysplasia and foci of microinvasion ( Fig. 2a ; arrow). Twelve weeks after termination of TPA treatment, the percentage of papillomas that progressed to malignancy was slightly increased in activin-overexpressing compared with wt and dnActRIB mice. Most importantly, the percentage of mice with malignant tumours was significantly higher in the groups of animals expressing the activin transgene ( Fig. 2b ). 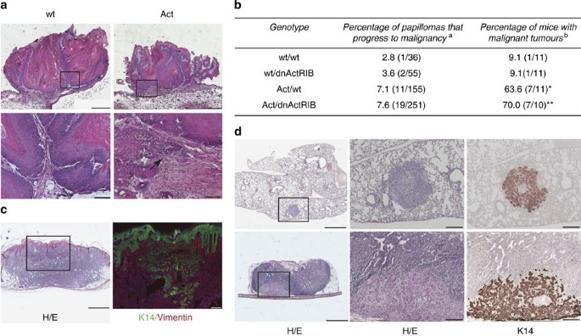Figure 2: Activin increases malignancy and metastatic spread of skin tumours. (a) Hematoxylin/eosin (H/E)-stained sections from papillomas 20 weeks after initiation. Local micro-invasive foci (arrow) were often observed in papillomas of Act mice (lower panel). Bars: 1,000 μm (top), 100 μm (bottom). Areas indicated by the box on the top pictures are shown at higher magnification on the bottom pictures. (b) Malignant conversion rate of tumours 32 weeks after initiation (experiment III).a()=number of carcinomas/total number of tumours.b()=number of mice with carcinomas/total number of mice.N=10 Act/dnActRIB mice,N=11 wt/wt, Act/wt, wt/dnActRIB mice; *P=0.0237 for Act/wt versus wt/wt, **P=0.0075 for Act/dnActRIB versus wt/wt (Fisher's exact test). (c) H/E staining (left) and double immunofluorescence for keratin (K)14 and vimentin (right) of a spindle cell variant of squamous cell carcinoma (SCC) in an Act mouse. Left bar: 1,000 μm; right bar: 200 μm. The area indicated by a box on the left picture is shown at higher magnification on the right picture. (d) Lung (top panel) and lymph node (bottom panel) metastases in carcinoma-bearing Act mice. Left and middle: H/E staining; right: K14 immunohistochemistry. Left bar: 1,000 μm; middle and right bars: 200 μm. Figure 2: Activin increases malignancy and metastatic spread of skin tumours. ( a ) Hematoxylin/eosin (H/E)-stained sections from papillomas 20 weeks after initiation. Local micro-invasive foci (arrow) were often observed in papillomas of Act mice (lower panel). Bars: 1,000 μm (top), 100 μm (bottom). Areas indicated by the box on the top pictures are shown at higher magnification on the bottom pictures. ( b ) Malignant conversion rate of tumours 32 weeks after initiation (experiment III). a ()=number of carcinomas/total number of tumours. b ()=number of mice with carcinomas/total number of mice. N =10 Act/dnActRIB mice, N =11 wt/wt, Act/wt, wt/dnActRIB mice; * P =0.0237 for Act/wt versus wt/wt, ** P =0.0075 for Act/dnActRIB versus wt/wt (Fisher's exact test). ( c ) H/E staining (left) and double immunofluorescence for keratin (K)14 and vimentin (right) of a spindle cell variant of squamous cell carcinoma (SCC) in an Act mouse. Left bar: 1,000 μm; right bar: 200 μm. The area indicated by a box on the left picture is shown at higher magnification on the right picture. ( d ) Lung (top panel) and lymph node (bottom panel) metastases in carcinoma-bearing Act mice. Left and middle: H/E staining; right: K14 immunohistochemistry. Left bar: 1,000 μm; middle and right bars: 200 μm. Full size image Histopathological analysis and immunostaining for keratins 14, 6, 10 and 13 revealed that most of the malignant tumours were squamous cell carcinomas (SCCs). Five out of 11 malignant tumours in Act/wt mice and 1 out of 19 in Act/dnActRIB mice had spindle-shaped tumour cells, showed vimentin immunoreactivity ( Fig. 2c ), and are likely to be a spindle cell variant of SCCs [18] . Four out of 9 activin-overexpressing mice with malignant tumours developed lung metastases ( Fig. 2d ), whereas this was not observed in wt mice. In experiment II, we collected inguinal and axillary lymph nodes 32 weeks after DMBA initiation. K14-positive metastatic nodules were observed in 3 out of 3 carcinoma-bearing Act-transgenic mice ( Fig. 2d ) and in 1 out of 2 wt mice with carcinomas. These results suggest that activin A not only accelerates tumourigenesis but also malignant progression of papillomas. Activin does not affect DMBA or TPA responsiveness To gain insight into the mechanisms underlying the enhanced tumourigenesis in Act mice, we analysed the skin before and following short-term treatment with DMBA and TPA. Consistent with the lack of obvious histological abnormalities in the back skin [8] , proliferation of keratinocytes and epidermal thickness were not altered in untreated Act mice ( Fig. 3a,b ). Several pro-inflammatory cytokines and chemokines were normally expressed ( Supplementary Fig. S2 ), and there was no inflammatory infiltrate in the skin (data not shown). 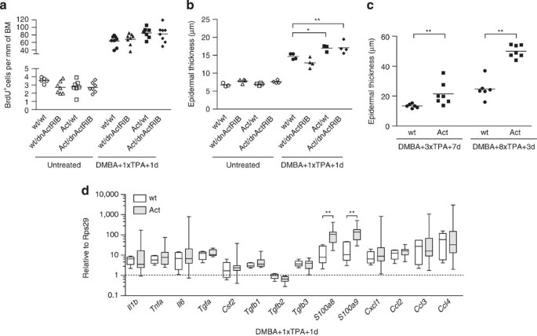Figure 3: Activin overexpression does not affect DMBA or TPA responsiveness. (a) Epidermal BrdU+cells per mm of basement membrane (BM) in untreated back skin or 1 day after the first TPA treatment. Scatter plot and mean values are shown;N=5–8 mice per group;n=6–23 microscopic fields of skin sections per mouse. (b) Epidermal thickness in untreated mice or 1 day after the first TPA treatment.N=3–4;n=6–13; *P≤0.05, **P≤0.01 (one-way ANOVA with Bonferroni post-test). (c) Epidermal thickness 7 days after the third TPA treatment or 3 days after the eighth TPA treatment.N=6–7;n=3–30; **P=0.0047 for 3×TPA, **P=0.0012 for 8×TPA (Mann–Whitney test). (d) RNA samples from back skin 1 day after the first TPA treatment were analysed for expression of pro-inflammatory cytokines and growth factors by quantitative reverse transcription PCR.N=5–10 mice per genotype.Rps29was used as reference. Box-and-whisker plot is depicted, with boxes showing median and 25th and 75th percentile, whiskers showing minimal and maximal values. **P=0.0047 forS100a8, **P=0.0027 forS100a9(Mann–Whitney test). Figure 3: Activin overexpression does not affect DMBA or TPA responsiveness. ( a ) Epidermal BrdU + cells per mm of basement membrane (BM) in untreated back skin or 1 day after the first TPA treatment. Scatter plot and mean values are shown; N =5–8 mice per group; n =6–23 microscopic fields of skin sections per mouse. ( b ) Epidermal thickness in untreated mice or 1 day after the first TPA treatment. N =3–4; n =6–13; * P ≤0.05, ** P ≤0.01 (one-way ANOVA with Bonferroni post-test). ( c ) Epidermal thickness 7 days after the third TPA treatment or 3 days after the eighth TPA treatment. N =6–7; n =3–30; ** P =0.0047 for 3×TPA, ** P =0.0012 for 8×TPA (Mann–Whitney test). ( d ) RNA samples from back skin 1 day after the first TPA treatment were analysed for expression of pro-inflammatory cytokines and growth factors by quantitative reverse transcription PCR. N =5–10 mice per genotype. Rps29 was used as reference. Box-and-whisker plot is depicted, with boxes showing median and 25th and 75th percentile, whiskers showing minimal and maximal values. ** P =0.0047 for S100a8 , ** P =0.0027 for S100a9 (Mann–Whitney test). Full size image We also could not detect alterations in the expression of several DMBA metabolizing or detoxifying enzymes, or in the proliferation rate of keratinocytes 24 h after DMBA treatment in Act versus wt mice ( Supplementary Fig. S2 ). One day after the first TPA treatment, we found a minor increase in keratinocyte proliferation and a slightly thicker epidermis in Act and Act/dnActRIB mice compared with control mice ( Fig. 3a,b; Supplementary Fig. S2 ). The difference in keratinocyte proliferation remained non-significant at later stages of TPA treatment ( Supplementary Fig. S2 ), but the difference in epidermal thickness increased continuously ( Fig. 3c ). The TPA-induced inflammatory response was not obviously altered by activin overexpression as determined by flow cytometry analysis of dermal single-cell suspensions (CD45 + leucocytes, Gr1 + CD11b + and Gr1 − CD11b + myeloid cells, CD3 + T cells and F4/80 + macrophages) ( Supplementary Fig. S3 ). Furthermore, several pro-inflammatory cytokines and chemokines were expressed at similar levels in TPA-treated skin of wt and Act mice ( Fig. 3d ). The only difference was the increased expression of S100A8 and A9 in Act mice, which most likely reflects an altered activation/differentiation state of the keratinocytes [17] . Several growth factors known to be induced by TPA and to contribute to TPA-induced tumour promotion [19] , [20] , [21] were expressed at similar levels in control and Act mice ( Fig. 3d ). In particular, expression of TGF-β1, β2 and β3 was not altered, suggesting that the observed phenotype is not due to differences in TGF-β expression ( Fig. 3d ). Finally, the number of blood vessels and the area of dermis covered by blood vessels 1d after the first TPA application as well as in papillomas collected after 20 TPA applications were similar in wt and Act mice ( Supplementary Fig. S3 ). Consistently, the expression levels of various angiogenesis-regulating factors were not altered by activin overexpression ( Supplementary Fig. S2 and S3 ). Loss of epidermal γδ T cells in TPA-treated Act mice Different subsets of T cells are either tumour-promotive or tumour-suppressive [22] , [23] . Dendritic epidermal T cells (DETCs) represent a subpopulation of unconventional, resident T cells expressing the γδ T-cell receptor (TcR) [24] . Remarkably, they kill skin-derived tumour cells in vitro and protect against different types of experimental skin tumours in vivo , including DMBA/TPA-induced papillomas and SCCs [25] , [26] . Immunofluorescence staining with pan-γδTcR antibodies revealed a severe depletion of γδ T cells in the non-tumourigenic epidermis of activin-overexpressing mice after 20 TPA applications ( Fig. 4a,b ), but not in untreated skin ( Fig. 4c ). Loss of these cells was dependent on TPA but not on DMBA ( Supplementary Fig. S4 ). A time course analysis revealed a continuous reduction in the number of epidermal but not of dermal γδ T cells in Act mice upon repeated TPA treatment ( Fig. 4d ; Supplementary Fig. S4 ). 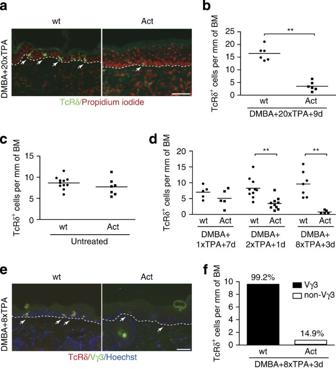Figure 4: Loss of epidermal γδ T cells in Act mice after TPA treatment. (a,b) Sections from non-tumourigenic skin of wt and Act mice after 20 TPA applications were stained with antibodies against TcRδ. Nuclei were counterstained with propidium iodide. (b) Quantification of epidermal TcRδ+cells per mm of basement membrane (BM).N=6 mice per genotype;n=6–16 microscopic fields of skin sections per mouse; **P=0.0022 (Mann–Whitney test). (c,d) Epidermal TcRδ+cells per mm of BM in untreated adult mice (c) and at different time points of TPA treatment (d). +1d, +3d and +7d indicate the number of days after TPA application.N=5–11;n=9–33; **P=0.0011 for DMBA+2×TPA+1d, **P=0.0025 for DMBA+8×TPA+3d (Mann–Whitney test). Scatter plot and mean values are shown in (b), (c) and (d). (e) Sections from back skin of wt and Act mice 3 days after the eighth TPA application were co-stained with antibodies against the pan-γδ TcR (TcRδ) and the Vγ3 variant of γδ TcR. Nuclei were counterstained with Hoechst. Arrows indicate TcRδ+cells. Representative micrographs are shown in (a) and (e). Arrows indicate TcRδ+cells. Bar: 50 μm. Dotted lines indicate dermal/epidermal border. (f) Epidermal TcRδ+cells and Vγ3+cells per mm of BM. Bar graph shows the mean number of TcRδ+cells per mm of BM, numbers above the columns indicate the corresponding percentage of Vγ3+cells among TcRδ+cells.N=7;n=3–13. Figure 4: Loss of epidermal γδ T cells in Act mice after TPA treatment. ( a , b ) Sections from non-tumourigenic skin of wt and Act mice after 20 TPA applications were stained with antibodies against TcRδ. Nuclei were counterstained with propidium iodide. ( b ) Quantification of epidermal TcRδ + cells per mm of basement membrane (BM). N =6 mice per genotype; n =6–16 microscopic fields of skin sections per mouse; ** P =0.0022 (Mann–Whitney test). ( c , d ) Epidermal TcRδ + cells per mm of BM in untreated adult mice ( c ) and at different time points of TPA treatment ( d ). +1d, +3d and +7d indicate the number of days after TPA application. N =5–11; n =9–33; ** P =0.0011 for DMBA+2×TPA+1d, ** P =0.0025 for DMBA+8×TPA+3d (Mann–Whitney test). Scatter plot and mean values are shown in ( b ), ( c ) and ( d ). ( e ) Sections from back skin of wt and Act mice 3 days after the eighth TPA application were co-stained with antibodies against the pan-γδ TcR (TcRδ) and the Vγ3 variant of γδ TcR. Nuclei were counterstained with Hoechst. Arrows indicate TcRδ + cells. Representative micrographs are shown in ( a ) and ( e ). Arrows indicate TcRδ + cells. Bar: 50 μm. Dotted lines indicate dermal/epidermal border. ( f ) Epidermal TcRδ + cells and Vγ3 + cells per mm of BM. Bar graph shows the mean number of TcRδ + cells per mm of BM, numbers above the columns indicate the corresponding percentage of Vγ3 + cells among TcRδ + cells. N =7; n =3–13. Full size image Epidermal γδ T cells uniformly express a TcR encoded by the Vγ3 gene segment [27] and display a characteristic dendritic morphology, whereas systemic γδ T cells in the lymphoid organs and lungs express the Vγ2 TcR [28] . Most of the γδ T cells remaining in Act animals after chronic TPA treatment lacked dendrites and had a lower TcRδ staining intensity ( Fig. 4a,e; Supplementary Fig. S4 ). Immunofluorescence staining revealed that four out of six activin-overexpressing mice completely lacked Vγ3 + DETCs in the epidermis after eight TPA applications ( Fig. 4e ). At this stage, only 14.9% of the remaining γδ T cells in the epidermis of Act mice, but >99% of these cells in wt mice were Vγ3 positive ( Fig. 4e,f ). Similar results were obtained for non-tumourigenic skin collected after 20 TPA applications, where Vγ3 + cells comprised >99% of all γδ T cells in wt mice versus 25% in Act mice. At the same time, a minor increase in Vγ2 + cells was observed in the epidermis of TPA-treated wt and Act animals ( Supplementary Fig. S4 ), whereas Vγ2 + cells were not found in the untreated epidermis of mice from both genotypes. Twelve weeks after termination of TPA application the number of TcRδ + cells remained very low in Act mice ( Supplementary Fig. S4 ). As precursors of γδ T cells are only present during embryonic development and can only populate the skin shortly after birth [29] , the depletion of DETCs is irreversible and the phenotype cannot be rescued by adoptive transfer of these cells. Epidermal γδ T cells express activin receptors Depletion of γδ T cells also occurred in Act/dnActRIB mice, suggesting that the effect is not mediated via keratinocytes ( Supplementary Fig. S4 ). To determine if activin can directly affect epidermal γδ T cells, we first analysed the expression of activin receptors by DETCs using RNA of fluorescence-activated cell (FACS)-sorted CD3 + TcRδ + cells from untreated epidermis of wt mice. The CD3 − TcRδ − population, consisting predominantly of keratinocytes and Langerhans cells, was used for comparison. DETCs expressed Acvr1, Acvr1c as well as Acvr2a and Acvr2b ( Fig. 5a ). Although we cannot exclude that the signal partially results from a minor contamination of the CD3 + TcRδ + fraction with K14-positive cells ( Fig. 5a ), the similar expression levels of most activin receptors in both populations strongly suggest that they are indeed expressed by DETCs. 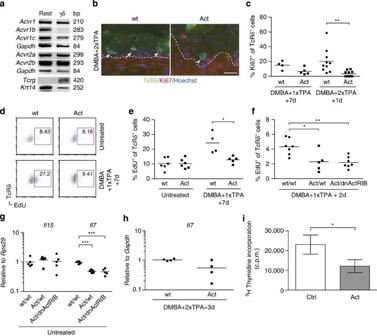Figure 5: Activin inhibits proliferation of epidermal γδ T cells. (a) CD3+TcRδ+(γδ T cells) and remaining cells (rest) were FACS sorted from the epidermis of three wt mice. RNA was analysed by reverse transcription PCR for expression of activin receptors,Gapdh, Krt14, and the γδ T cell receptor (Tcrg). (b,c) Sections from TPA-treated back skin of wt and Act mice stained for TcRδ and Ki67. (b) The dotted line indicates the epidermal–dermal border. Arrows and arrowheads indicate Ki67+TcRδ+or Ki67−TcRδ+cells, respectively. Bar: 25 μm. (c) Percentage of Ki67+cells among TcRδ+cells 7 days after the first or 1 day after the second TPA application.N=4–10 mice per genotype;n=17–22 microscopic fields of skin sections per mouse; **P=0.0019 (Mann–Whitney test). (d) Untreated or DMBA/TPA-treated mice were injected with EdU twice a day for 7 days. Epidermal single-cell suspensions were analysed for EdU incorporated in TcRδ+cells by flow cytometry. Representative pseudo-colour plots are shown (gated on viable TcRδ+cells). The percentage of EdU+cells among the TcRδ+cells is indicated. Data shown are representative of at least four independent analyses. (e,f) The percentage of EdU+cells among the TcRδ+cells was quantified by flow cytometry before and at different time points after TPA treatment. (e) EdU was injected twice a day for 7 days;N=4–6; *P=0.0159 (Mann–Whitney test). (f) EdU was injected twice a day for 2 days;N=5–7; *P≤0.05; **P≤0.01 (one-way ANOVA with Bonferroni post-test). (g,h) RNA samples from trypsin-separated epidermis from untreated mice (g) or from mice after the second TPA application (h) were analysed for expression ofIl15andIl7by quantitative reverse transcription PCR usingRps29orGapdhas reference. Expression in one of the wt mice was arbitrarily set to 1.N=4–5; ***P≤0.001 (one-way ANOVA with Bonferroni post-test). Scatter plot and mean values are shown in (c), (e), (f), (g) and (h). (i) Vγ3+Thy1.2+cells were FACS sorted and cultured for 48 h with immobilized anti-CD3 antibodies (0.1 μg ml−1) in the absence (ctrl) or presence of 50 ng ml−1activin A (Act).3H-thymidine incorporation assay was performed in quadruplicates. Data are representative of two independent experiments; mean values±s.d. are shown; *P=0.0286 (Mann–Whitney test). Figure 5: Activin inhibits proliferation of epidermal γδ T cells. ( a ) CD3 + TcRδ + (γδ T cells) and remaining cells (rest) were FACS sorted from the epidermis of three wt mice. RNA was analysed by reverse transcription PCR for expression of activin receptors, Gapdh, Krt14 , and the γδ T cell receptor ( Tcrg ). ( b , c ) Sections from TPA-treated back skin of wt and Act mice stained for TcRδ and Ki67. ( b ) The dotted line indicates the epidermal–dermal border. Arrows and arrowheads indicate Ki67 + TcRδ + or Ki67 − TcRδ + cells, respectively. Bar: 25 μm. ( c ) Percentage of Ki67 + cells among TcRδ + cells 7 days after the first or 1 day after the second TPA application. N =4–10 mice per genotype; n =17–22 microscopic fields of skin sections per mouse; ** P =0.0019 (Mann–Whitney test). ( d ) Untreated or DMBA/TPA-treated mice were injected with EdU twice a day for 7 days. Epidermal single-cell suspensions were analysed for EdU incorporated in TcRδ + cells by flow cytometry. Representative pseudo-colour plots are shown (gated on viable TcRδ + cells). The percentage of EdU + cells among the TcRδ + cells is indicated. Data shown are representative of at least four independent analyses. ( e , f ) The percentage of EdU + cells among the TcRδ + cells was quantified by flow cytometry before and at different time points after TPA treatment. ( e ) EdU was injected twice a day for 7 days; N =4–6; * P =0.0159 (Mann–Whitney test). ( f ) EdU was injected twice a day for 2 days; N =5–7; * P ≤0.05; ** P ≤0.01 (one-way ANOVA with Bonferroni post-test). ( g , h ) RNA samples from trypsin-separated epidermis from untreated mice ( g ) or from mice after the second TPA application ( h ) were analysed for expression of Il15 and Il7 by quantitative reverse transcription PCR using Rps29 or Gapdh as reference. Expression in one of the wt mice was arbitrarily set to 1. N =4–5; *** P ≤0.001 (one-way ANOVA with Bonferroni post-test). Scatter plot and mean values are shown in ( c ), ( e ), ( f ), ( g ) and ( h ). ( i ) Vγ3 + Thy1.2 + cells were FACS sorted and cultured for 48 h with immobilized anti-CD3 antibodies (0.1 μg ml −1 ) in the absence (ctrl) or presence of 50 ng ml −1 activin A (Act). 3 H-thymidine incorporation assay was performed in quadruplicates. Data are representative of two independent experiments; mean values±s.d. are shown; * P =0.0286 (Mann–Whitney test). Full size image Activin inhibits γδ T cell proliferation We next determined the reason underlying the loss of DETCs upon TPA treatment. Although the K14 promoter is active in thymic epithelial cells [30] , the number of the foetal thymic precursors of DETCs was not obviously affected in Act mice ( Supplementary Fig. S5 ), and developmental abnormalities are therefore unlikely. This is also reflected by the normal number and morphology of DETCs in untreated skin of Act mice ( Fig. 4c ). Furthermore, loss of DETCs did not result from their emigration to the draining lymph nodes induced by stressed keratinocytes [31] , as the number of TcRδ + cells present in the skin-draining lymph nodes of TPA-treated skin was similar in wt and transgenic mice ( Supplementary Fig. S5 ). Apoptosis of DETC was excluded by staining of sections from TPA-treated skin for cleaved caspase-3 or by TUNEL. In vitro , addition of 12.5 or 50 ng ml −1 activin A to resting or stimulated DETC 7-17 cells or freshly isolated epidermal γδ T cells did not affect their survival as assessed by flow cytometry analysis of 7-AAD exclusion or by annexin V/propidium iodide staining (data not shown). Finally, we determined if activin affects proliferation of DETCs using Ki67 immunofluorescence staining of skin sections prepared 7 days after the first TPA or 1 day after the second TPA application. In all, 20% of the TcRδ + cells in the epidermis of wt mice, but only 3.5% in Act mice expressed Ki67 ( Fig. 5b,c ). To verify this finding, we labelled proliferating cells in vivo with 5-ethynyl-2′-deoxyuridine (EdU), and subsequently analysed the percentage of EdU-positive TcRδ + cells using flow cytometry. Whereas γδ T cell proliferation was similar in untreated skin of mice from both genotypes, proliferation of DETCs increased in response to TPA in wt mice, but not in Act or Act/dnActRIB mice ( Fig. 5d–f ). Analysis of the DETC growth and survival factors interleukin (IL)-7 and IL-15 [32] , [33] revealed that activin did not affect IL-15 expression. However, IL-7 mRNA levels were reduced by ∼ 50% in non-treated skin and after the second TPA application in Act and Act/dnActRIB animals ( Fig. 5g,h ). In addition, activin directly reduced the proliferation rate of primary DETCs in the presence of suboptimal concentrations of anti-CD3 antibodies ( Fig. 5i ). Therefore, activin seems to suppress DETC proliferation through direct and indirect mechanisms during chronic TPA treatment when these cells have to be amplified to maintain an appropriate number in the hyperproliferative epidermis, which has a high turnover. Activin increases epidermal αβ T cells and Langerhans cells The loss of γδ T cells phenocopies the situation seen in γδ T-cell-deficient mice and thus provides a likely mechanistic explanation for the enhanced carcinogenesis in activin-overexpressing mice. To determine if additional types of immune cells can further enhance the pro-tumourigenic effect of activins, we first analysed αβ T cells that promoted malignant conversion in the model of chemically induced skin carcinogenesis [26] . There was no significant difference in the number of αβ T cells in the dermis of TPA-treated skin ( Supplementary Fig. S5 ). However, the number of αβ T cells infiltrating the epidermis during DMBA/TPA-induced tumourigenesis was significantly higher in activin-overexpressing mice ( Fig. 6a,b ). Thus, lack of γδ T cells is likely to act in concert with the accumulation of αβ T cells in the promotion of carcinogenesis. 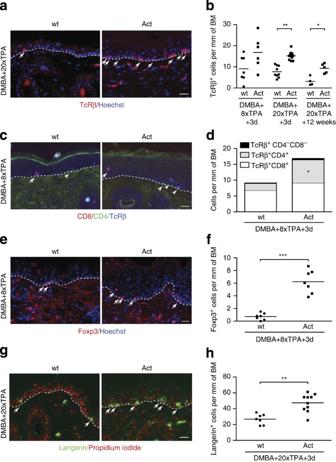Figure 6: Accumulation of αβ T cells and Langerhans cells in the epidermis of activin-overexpressing mice. (a,b) Sections from back skin at different time points of TPA treatment stained with TcRβ antibodies. (a) Arrows indicate TcRβ+cells. (b) TcRβ+cells per mm of basement membrane (BM).N=4–11 mice per group;n=3–25 microscopic fields of skin sections per mouse; *P=0.0159; **P=0.0022 (Mann–Whitney test). (c,d) Sections from back skin after eight TPA applications stained with antibodies against CD8, CD4 and TcRβ. (c) Arrows and arrowheads indicate CD8+or CD4+cells, respectively. (d) Different subpopulations of T cells per mm of BM.N=6–7;n=4–24; mean values are shown; *P=0.01 for comparison of TcRβ+CD4+cells between wt and Act mice (Mann–Whitney test). (e,f) Sections from back skin after eight TPA applications stained with Foxp3 antibodies. (e) Arrows indicate Foxp3+cells. (f) Epidermal Foxp3+cells per mm of BM.N=7;n=6–25; ***P=0.0006 (Mann–Whitney test). (g,h) Sections from back skin after 20 TPA applications stained with langerin antibodies. (g) Arrows indicate langerin+cells. (h) Langerin+cells per mm of BM.N=7–10;n=3–25; **P=0.0012 (Mann–Whitney test). Representative sections are shown in (a), (c), (e) and (g), and the dermal–epidermal border is indicated by dotted lines. Nuclei were counterstained with Hoechst (a), (c), and (e) or propidium iodide (g). Bars: 25 μm. Scatter plots and mean values are shown in (b), (f) and (h). Figure 6: Accumulation of αβ T cells and Langerhans cells in the epidermis of activin-overexpressing mice. ( a , b ) Sections from back skin at different time points of TPA treatment stained with TcRβ antibodies. ( a ) Arrows indicate TcRβ + cells. ( b ) TcRβ + cells per mm of basement membrane (BM). N =4–11 mice per group; n =3–25 microscopic fields of skin sections per mouse; * P =0.0159; ** P =0.0022 (Mann–Whitney test). ( c , d ) Sections from back skin after eight TPA applications stained with antibodies against CD8, CD4 and TcRβ. ( c ) Arrows and arrowheads indicate CD8 + or CD4 + cells, respectively. ( d ) Different subpopulations of T cells per mm of BM. N =6–7; n =4–24; mean values are shown; * P =0.01 for comparison of TcRβ + CD4 + cells between wt and Act mice (Mann–Whitney test). ( e , f ) Sections from back skin after eight TPA applications stained with Foxp3 antibodies. ( e ) Arrows indicate Foxp3 + cells. ( f ) Epidermal Foxp3 + cells per mm of BM. N =7; n =6–25; *** P =0.0006 (Mann–Whitney test). ( g , h ) Sections from back skin after 20 TPA applications stained with langerin antibodies. ( g ) Arrows indicate langerin + cells. ( h ) Langerin + cells per mm of BM. N =7–10; n =3–25; ** P =0.0012 (Mann–Whitney test). Representative sections are shown in ( a ), ( c ), ( e ) and ( g ), and the dermal–epidermal border is indicated by dotted lines. Nuclei were counterstained with Hoechst ( a ), ( c ), and ( e ) or propidium iodide ( g ). Bars: 25 μm. Scatter plots and mean values are shown in ( b ), ( f ) and ( h ). Full size image Characterization of the subpopulations of αβ T cells revealed that the number of epidermal CD8 + cells was only slightly increased in transgenic animals, whereas significantly more CD4 + cells had infiltrated the epidermis of Act mice after eight TPA treatments ( Fig. 6c,d ). Staining with an antibody against the regulatory T cell (Treg) marker Foxp3 revealed a significant increase in these immunosuppressive cells in the epidermis of Act animals after chronic TPA treatment ( Fig. 6e,f ), but not in the dermis ( Supplementary Fig. S5 ). We found a significant increase in the number of Langerhans cells in DMBA/TPA-treated Act mice ( Fig. 6g,h ). The percentage of langerin-positive cells that also expressed the activation marker CD86 was similar in wt and Act mice, suggesting that activation of Langerhans cells is not obviously impaired ( Supplementary Fig. S6 ). As Langerhans cells promote DMBA/TPA-induced skin carcinogenesis [34] , they are likely to further contribute to the pro-tumourigenic phenotype in Act mice. Taken together, our results demonstrate that activin induces a pro-tumourigenic immune cell response, which involves different types of epidermal T cells and Langerhans cells. Activin is overexpressed in human skin carcinomas Finally, we addressed the role of endogenous activin in skin carcinogenesis in mice and humans. Consistent with a role of endogenous activin in skin carcinogenesis, activin βA ( Inhba ) mRNA levels were slightly upregulated after short-term TPA treatment and were almost 100-fold increased in the papillomas of wt mice compared with untreated skin ( Supplementary Fig. S7 ). Most importantly, we found a strong increase in the levels of activin βA mRNA in human basal cell carcinomas (BCC) and even more in SCC samples as compared with normal skin ( Fig. 7a ), whereas follistatin RNA levels were similar in normal and tumourigenic skin ( Fig. 7b ). Immunohistochemical staining of sections from human SCCs with an activin A-specific antibody revealed that activin is expressed by keratinocytes of the tumour as well as in the adjacent epidermis ( Fig. 7c–e ). Epidermal staining was also seen in normal skin ( Fig. 7f ). In addition, staining was observed in blood vessels of normal skin and in particular in the enlarged tumour vessels ( Fig. 7d,e ). This finding reflects the importance of our data for human skin carcinogenesis. 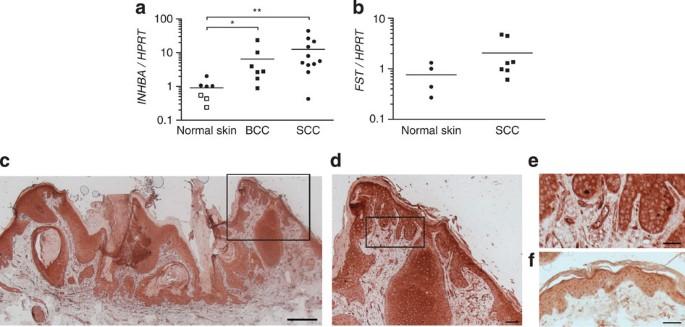Figure 7: Activin is overexpressed in human skin carcinomas. (a) RNA samples from normal human skin, basal cell carcinomas (BCCs) and SCCs were analysed for expression of activin βA (INHBA) by quantitative reverse transcription PCR. Hypoxanthine-guanine phosphoribosyl-transferase(HPRT)was used as a reference. Expression levels in one of the normal skin samples were set to 1. Closed and open squares represent values from normal skin collected from the edge of tumours or from healthy adult volunteers, respectively.N=7 normal skin samples;N=7 BCC samples;N=11 SCC samples; *P=0.0111, **P=0.0038 (Mann–Whitney test). (b) RNA samples from normal human skin and SCCs were analysed for expression of follistatin(FST)by quantitative reverse transcription PCR.HPRTwas used as a reference.N=4 normal skin samples;N=7 SCC samples. Scatter plot and median values are shown in (a) and (b). (c–f) Sections of human SCCs (c–e) and normal skin (f) were stained with an activin A antibody and counterstained with hematoxylin. The areas indicated by the box in (c) and (d) are shown at high magnification in (d) and (e), respectively. Note the expression of activin in the tumour cells and in blood vessels. Bar: 500 μm (c), 100 μm (d) or 50 μm (e,f). Figure 7: Activin is overexpressed in human skin carcinomas. ( a ) RNA samples from normal human skin, basal cell carcinomas (BCCs) and SCCs were analysed for expression of activin βA ( INHBA ) by quantitative reverse transcription PCR. Hypoxanthine-guanine phosphoribosyl-transferase (HPRT) was used as a reference. Expression levels in one of the normal skin samples were set to 1. Closed and open squares represent values from normal skin collected from the edge of tumours or from healthy adult volunteers, respectively. N =7 normal skin samples; N =7 BCC samples; N =11 SCC samples; * P =0.0111, ** P =0.0038 (Mann–Whitney test). ( b ) RNA samples from normal human skin and SCCs were analysed for expression of follistatin (FST) by quantitative reverse transcription PCR. HPRT was used as a reference. N =4 normal skin samples; N =7 SCC samples. Scatter plot and median values are shown in ( a ) and ( b ). ( c – f ) Sections of human SCCs ( c – e ) and normal skin ( f ) were stained with an activin A antibody and counterstained with hematoxylin. The areas indicated by the box in ( c ) and ( d ) are shown at high magnification in ( d ) and ( e ), respectively. Note the expression of activin in the tumour cells and in blood vessels. Bar: 500 μm ( c ), 100 μm ( d ) or 50 μm ( e , f ). Full size image In this study, we provide a new molecular link between wound healing and cancer: The major orchestrator of wound repair, the growth and differentiation factor activin, was identified as a potent pro-tumourigenic factor in the skin. Remarkably, blocking activin receptor signalling in keratinocytes revealed that the pro-tumourigenic effect is predominantly mediated via the stroma. This was further supported by the similar proliferation rate of keratinocytes in wt and Act mice in vivo and in vitro (M.A., M.M. and S.W unpublished results). Although activin can have both pro- and anti-inflammatory properties [4] , we did not find significant alterations in various inflammatory parameters in normal or DMBA/TPA-treated back skin of activin-transgenic mice. Similarly, activin demonstrated pro- [35] or anti-angiogenic [36] properties in different systems. However, our results suggest that the pro-tumourigenic function of activin in the skin does not result from its effect on angiogenesis. By contrast, activin strongly affected cells involved in tumour immunosurveillance. In particular, DETCs were depleted in TPA-treated skin of Act mice. As these cells have a tumour-suppressive function [25] , [26] , their loss is likely to result in reduced clearance of stressed/transformed keratinocytes and a subsequent increase in tumour formation as demonstrated previously for γδ T-cell-deficient mice [25] and here for our activin-transgenic animals. As the underlying mechanism, we identified a potent growth inhibitory effect of activin for DETCs. The results obtained with double-transgenic mice suggest that this phenomenon is not mediated via activin-induced alterations of keratinocytes, but rather involves a direct action of activin on DETCs or is mediated via other stromal cells. The first hypothesis is supported by the expression of activin receptors by DETCs in vivo and the inhibition of primary epidermal γδ T-cell proliferation by activin in vitro . Growth inhibition of DETCs is likely to be further enhanced in vivo through reduced expression of IL-7 in Act mice. As IL-7 functions as a homoeostatic signal, preventing atrophy and sustaining the basal rate of metabolism in T cells [37] , its reduction in activin-overexpressing mice could result in a dampened metabolic rate of DETCs, inhibiting proliferation after chronic stimulation by TPA. Apart from targeting the tumours directly, DETCs were also suggested to reduce the potential of αβ T cells to promote tumourigenesis [38] . Therefore, lack of γδ T cells is likely to act in concert with the accumulation of αβ T cells in the promotion of carcinogenesis. The increase in epidermal αβ T cells also provides a likely explanation for the enhanced malignant progression of existing tumours, as these cells also promoted tumour progression in TcRδ −/− mice [26] . Consistent with the recently identified role of activin in induction of Tregs [39] , [40] , we found a significant accumulation of Foxp3 + cells in the epidermis of TPA-treated activin-overexpressing mice. Interestingly, Foxp3 + cells also infiltrate human SCCs and are thought to at least in part mediate the evasion of the immune response by these tumours [41] . Finally, we found a significant increase in the number of Langerhans cells in TPA-treated skin of activin-overexpressing mice. This finding is consistent with the reduction in the number of Langerhans cells in follistatin-overexpressing mice [42] and with the activin A-induced Langerhans cell differentiation in vitro and in human skin samples [43] . As Langerhans cells promote DMBA/TPA-induced skin carcinogenesis [34] , they are likely to further contribute to the pro-tumourigenic phenotype in Act mice. In the future, it will be interesting to determine if there is a possible contribution of these and additional immune cells in the response to activin. Interesting candidates are macrophages that differentiate towards the immuno-suppressive and tumour-promotive M2 phenotype in response to activin [44] , as well as dendritic cells and natural killer cells that are functionally affected by activin [45] , [46] . The functional data obtained with our mouse models are likely to be important for the human situation, as we found a strong increase in activin A expression in human BCCs and in particular in SCCs. In the future, it will be important to determine if the enhanced expression of activin seen in these tumours correlates with abnormalities in the T-cell repertoire in the affected patients. Although epidermal γδ T cells are much more abundant in murine skin compared with human skin, they contribute to efficient wound repair in humans [47] . In some patients, the percentage of γδ T cells among epidermal T cells can be up to 20%. In addition, functional findings for murine epidermal T cells have also been applicable for human epidermal-resident T cells [47] , [48] . Therefore, they may well contribute to skin carcinogenesis, an issue that should be explored in the future. Such studies will also reveal if enhanced expression of activin affects anti-tumour immunity in humans, resulting in more malignant tumours and metastatic spread. The recently observed upregulation of activin expression in keratinocytes of human oral SCCs and the correlation of activin overexpression with poor prognosis strongly support this hypothesis [49] . Thus, targeting of activin or its downstream mediators may emerge as a novel approach for the treatment of carcinomas that overexpress this factor. As activin antagonists were recently shown to reverse cancer cachexia and muscle wasting [50] and cancer-induced bone destruction [51] , [52] in animal models, it may well be that targeting activin action could inhibit tumour growth and progression, and at the same time prevent cancer-induced morbidity. Animal experiments Mice were housed under optimal hygiene conditions and maintained according to Swiss animal protection guidelines. All procedures with mice were approved by the local veterinary authorities of Zurich or Lausanne, Switzerland. Genotyping of genetically modified mice is described in the Supplementary Methods . For chemical skin carcinogenesis, 25 μg of DMBA (Sigma) dissolved in acetone was applied on the back skin of 8–10-week-old female mice 2 days after shaving. One week later, 5 μg (CD1 background) or 7.5 μg (mixed background) of TPA (Sigma) in acetone was applied weekly for 20 weeks. We used a higher dosage of TPA for the animals of a mixed genetic background, as the parental strains of dnActRIB mice (C57BL/6 and DBA/2) are relatively resistant to chemically induced skin carcinogenesis [53] . A summary of all carcinogenesis experiments with the concentrations of DMBA and TPA used is presented in Table 1 . Tumour number and size were documented bi-weekly. After 20 weeks of TPA treatment, half of the animals of each genotype were killed. Biopsies of non-tumourigenic back skin and all tumours with at least 2 mm diameter were used for histology, immunohistochemistry or RNA isolation. TPA treatment was stopped after 20 weeks and tumour observation was continued until the mice started to develop ulcerated tumours (30–40 weeks after initiation). All large and/or ulcerated tumours were collected for histopathological analysis by three independent investigators with expertize in cutaneous histopathology. Lungs and lymph nodes were embedded in paraffin, and every 7–10th section was stained with hematoxylin/eosin (H/E) and examined for the presence of metastatic nodules. Immunofluorescence and immunohistochemical analysis For preparation of frozen sections, tissue samples were immediately frozen in tissue freezing medium (Leica Microsystems). For preparation of paraffin sections, they were either fixed in 95% ethanol/1% acetic acid or in 4% paraformaldehyde. Cryosections (4 or 7 μm) were fixed with ice-cold methanol for 10 min. Paraffin sections were deparaffinized through incubation in xylene and subsequently in a graded series of ethanol. Sections were then blocked with 3% bovine serum albumin (BSA) and incubated with the primary antibody, followed by a fluorochrome-labelled secondary antibody. For immunohistochemistry, sections were incubated with biotinylated secondary antibodies and developed using the Vectastain ABC kit and 3-amino-9-ethylcarbazole (AEC) or 3,3′-diaminobenzidine (DAB) peroxidase substrate kits (Vector Laboratories). The antibodies used are listed in Supplementary Table S1 . For activin A immunohistochemistry, formalin-fixed paraffin sections were deparaffinized and incubated for 45 min at 98 °C in 0.5 M ethylenediaminetetraacetic acid pH 8 in a water bath for antigen retrieval. Endogenous peroxidase activity was blocked by incubation in 3–4% H 2 O 2 , while unspecific binding sites were blocked by a 1-h incubation at room temperature in 12% BSA, 0.1% Tween 20, 0.1% NP40 in phosphate-buffered saline. Subsequently, the sections were incubated overnight at 4 °C with the primary antibody, followed by a 1-h incubation at room temperature with a horse radish peroxidase (HRP)-conjugated secondary antibody. The anti-rabbit poly-HRP-IgG polymer from the Bond Polymer Refine Detection System (Leica Microsystems) was used for enhancement of the signal. The substrate chromogen, DAB, was used for detection of the complex. Sections were counterstained with hematoxylin. Stained sections were photographed using an Imager.A1 microscope equipped with an Axiocam Mrm camera and enhanced-contrast Plan-Neofluor objectives (10×/0.3 NA, 20×/0.5 NA; all from Carl Zeiss, Inc.). Axiovision 4.6 software (Carl Zeiss, Inc) was used for data acquisition. BrdU incorporation assay Mice were injected intraperitoneally with 250 mg kg −1 BrdU 2 h before killing. Samples were fixed in 95% ethanol/1% acetic acid, and embedded in paraffin. BrdU-positive cells were detected with a horseradish peroxidase-conjugated monoclonal antibody against BrdU (Roche), and visualized with 0.05% DAB/0.005% H 2 O 2 . Counterstaining was performed with H/E. TUNEL assay Apoptosis on tissue sections was analysed using the In situ Cell Death Detection Kit (Roche) according to the manufacturer's instructions. RNA isolation and quantitative reverse transcription PCR Total RNA was isolated using the RNeasy Fibrous Tissue Mini Kit or the RNeasy Midi Kit (Qiagen) according to the manufacturer's instructions, including a DNase treatment step (Promega). cDNA was synthesized using the iScript kit (Bio-Rad Laboratories). Relative gene expression was determined using the Roche LightCycler 480 SYBR Green system (Roche). The gene-specific primers used are listed in Supplementary Table S2 . Isolation of cells for flow cytometry Single-cell suspensions of epidermal cells were prepared as described previously [54] . Disaggregated epidermal cells were filtered through a 70-μm nylon cell strainer (BD Pharmingen), centrifuged at 1,200 rpm at 4 °C for 10 min and resuspended in FACS buffer (phosphate-buffered saline, 0.2% BSA and 5 mM ethylenediaminetetraacetic acid). Dermis was cut into small pieces, and incubated for 45 min at 37 °C under continuous shaking in DMEM containing 2.5 mg ml −1 collagenase II (Worthington), 2.5 mg ml −1 collagenase IV (Invitrogen), 0.5 mg ml −1 DNase I and 1 mg ml −1 hyaluronidase (Worthington). Thymi were mechanically disaggregated and filtered through a 70-μm nylon cell strainer. Lymph nodes were incubated for 30 min at 37 °C under continuous shaking in DMEM containing 5 mg ml −1 of collagenase IV (Invitrogen). Disaggregated dermal cells were treated as described for epidermal cells. Flow cytometry Cells were incubated for 10 min at 4 °C with rat anti-mouse CD16/CD32 monoclonal antibody (clone 2.4G2, BD Biosciences) to prevent non-specific antibody binding, followed by a 30-min incubation at 4 °C with directly labelled specific antibodies ( Supplementary Table S3 ). After washing with FACS buffer, 7-AAD (BD Biosciences) was added to discriminate between viable and dead cells. Data acquisition was performed using a FACS Calibur equipped with CellQuestPro software (BD Biosciences) and analysis was done using FlowJo software (Tree Star Inc.). FACS sorting and reverse transcription PCR Epidermal cells were isolated, stained with antibodies as described above, and FACS sorted using a FACS Aria Cell Sorter (BD Biosciences). RNA was isolated from the sorted cells using the RNeasy Micro Kit (Qiagen), and cDNA was generated using the High-Capacity cDNA Reverse Transcription Kit (Applied Biosystems) according to the manufacturers' instructions. DETC culture The 7–17 DETC line was grown in RPMI 1640 medium supplemented with 10% FCS, 25 mM HEPES, 100 U penicillin 100 μg −1 streptomycin, 2 mM glutamine, 100 μM non-essential amino acids, 1 mM sodium pyruvate, 50 μM 2-mercaptoethanol and 20 U ml −1 of recombinant human IL-2. Cells were restimulated every 4–5 weeks overnight with 5 μg/ml −1 of concanavalin A and were allowed to rest for 2 weeks before use in assays. For isolation of primary DETCs, skin was incubated on 0.3% trypsin for 2–2.5 h at 37 °C, and the epidermis was separated from the dermis. Epidermis was incubated for 10 min in 0.3% trypsin at 37 °C. The epidermal preparation was enriched for live cells by centrifugation over lympholyte M, and cells recovered from the interface were cultured as described above, with the exception that the medium contained 10 U ml −1 of IL-2. Survival and proliferation experiments were performed with recombinant activin A (R&D Systems). Survival of DETCs was assessed by 7-AAD exclusion or annexin V/propidium iodide staining. For proliferation analysis, Vγ3 + Thy1.2 + cells were FACS sorted and subsequently cultured in the presence of immobilized anti-CD3 antibodies (BD Biosciences, clone 500A2, 0.1 μg ml −1 ), with or without activin A. They were pulsed with 0.5μ Ci 3 H-thymidine, harvested 18 h later onto glass fibre filters, and counts were detected in a scintillation counter. EdU incorporation assay EdU (Invitrogen) was injected intraperitoneally twice a day (100 μg per mouse). Incorporated EdU was analysed in epidermal single-cell suspensions by flow cytometry using the Click-iT EdU Flow Cytometry Assay Kit (Invitrogen). The LIVE/DEAD Fixable Dead Cell Stain Kit (Invitrogen) was used to discriminate between live and dead cells. Human skin biopsies Normal human skin and skin cancer samples were obtained anonymously from the Departments of Dermatology, University Hospitals of Lausanne and Zurich (in the context of the biobank project), approved by the local and cantonal Research Ethics Committees. Normal skin was from healthy adult volunteers or from the edges of skin tumours. BCC or SCC was diagnosed by experienced pathologists. Informed consent for research was obtained before routine diagnostic services. All samples included the dermis and the epidermis. Statistical analysis Statistical analysis was performed using the GraphPad Prism version 5.0 for Mac OS X (GraphPad Software). For analysis of tumour incidence, comparison of the curves showing the mice with tumours was performed using log-rank χ 2 test. Tumour multiplicity was analysed using two-way repeated measures analysis of variance (ANOVA). Malignant conversion rate and the percentage of mice with malignant tumours were analysed by Fisher's exact test. Mann–Whitney test was used for comparing two groups of data; ANOVA test was used for comparing three or more groups. * P ≤0.05, ** P ≤0.01 and *** P ≤0.001. Differences between groups that were not labelled with asterisks were non-significant. How to cite this article: Antsiferova, M. et al . Activin enhances skin tumourigenesis and malignant progression by inducing a pro-tumourigenic immune cell response. Nat. Commun. 2:576 doi: 10.1038/ncomms1585 (2011).